Synergistic roles for lipids and proteins in the permanent adhesive of barnacle larvae Thoracian barnacles rely heavily upon their ability to adhere to surfaces and are environmentally and economically important as biofouling pests. Their adhesives have unique attributes that define them as targets for bio-inspired adhesive development. With the aid of multi-photon and broadband coherent anti-Stokes Raman scattering microscopies, we report that the larval adhesive of barnacle cyprids is a bi-phasic system containing lipids and phosphoproteins, working synergistically to maximize adhesion to diverse surfaces under hostile conditions. Lipids, secreted first, possibly displace water from the surface interface creating a conducive environment for introduction of phosphoproteins while simultaneously modulating the spreading of the protein phase and protecting the nascent adhesive plaque from bacterial biodegradation. The two distinct phases are contained within two different granules in the cyprid cement glands, implying far greater complexity than previously recognized. Knowledge of the lipidic contribution will hopefully inspire development of novel synthetic bioadhesives and environmentally benign antifouling coatings. The ocean is a complex mixture of dissolved ions and organic macromolecules with a pH and ionic strength that vary significantly with geographical location. Over the past 500 million years or so, sessile marine invertebrates have evolved diverse adhesion mechanisms to suit the varied assortment of materials that constitute their settlement substrata, including rocks of differing chemistry, plants and the surfaces of other animals. Performing the complex chemistry of adhesion in such a variable environment is not a trivial matter, yet adhesion to surfaces is routine for most sessile marine invertebrates and it is unusual to find a naturally occurring surface to which barnacles, for example, cannot attach. Indeed, both generalist barnacle species and those that are highly surface-specific have evolved mechanisms that facilitate tenacious adhesion, under particularly hostile conditions, to surfaces that differ significantly in terms of roughness, chemistry, elastic modulus, surface energy and charge [1] . In addition, organic materials released into the ocean, particularly to a surface, quickly become a target for bacteria and may be damaged by digestive enzymes and other extracellular polymeric substances. Since many barnacles settle readily onto biogenic surfaces and persist there for years, their adhesives must have evolved in a long-running ‘arms race’, both against bacteria and organisms that need to remain clear of epibionts [2] . The bioadhesive systems of barnacles and other sessile marine invertebrates have in fact become so effective that most living surfaces that resist colonization do so via toxic means [3] , grooming [4] or by sloughing [5] . It is imperative that surface-colonizing forms of marine invertebrates remain securely attached to a chosen substratum during metamorphosis and growth; dislodgement usually equates to death. To be effective, their adhesives must overcome the adverse physical conditions at hydrated interfaces as well as the presence of biofilm. In light of these challenges, the adhesive used by the barnacle cypris larva (or cyprid) during permanent attachment to a surface presents an interesting model for the development of synthetic adhesives with wide-ranging applications. The adhesives of marine organisms, and of barnacles in particular, are therefore of significant commercial interest for novel biomedical adhesives and implants, being already optimized for conditions akin to those in the human body. However, improved knowledge of their mechanisms of action will also inform the design of novel coating technologies to combat marine biofouling [6] . Ship hull fouling costs between $180 and $260 million per annum for the US Navy [7] alone and contributes to a loss in cruising efficiency of up to 86% for a typical Navy ship [8] . The economic and environmental consequences of fouling, including higher fuel bills, translocation of invasive species and greenhouse gas emissions, are also becoming increasingly high profile as environmental restrictions on the use of antifouling biocides are tightened. Cypris larvae adhere permanently to surfaces using an adhesive exuded from large, paired glandular structures located posterior to their compound eyes [9] ( Fig. 1a,b ). This material (the cyprid permanent adhesive or, historically, ‘cement’) is apparently unrelated to the cyprid temporary adhesive (used during surface exploration before settlement [10] ) and similarity to the adult barnacle adhesive remains to be thoroughly investigated. The permanent adhesive (or ‘cement’) glands were described originally by Darwin [11] and details of the morphology, biochemistry and mechanism of action of the cyprid adhesive system have advanced relatively slowly since. The adhesives of barnacles have long been known to differ from those of other sessile marine invertebrates [12] . Whereas mussels [13] , tubeworms [14] and echinoderms [15] , for example, rely on DOPA-rich or poly-phosphorylated peptides that are stored separately in glandular structures, crosslinking covalently upon release for adhesion, adult barnacle cement components are released from single cells and the sequence of release and the curing mechanism(s) remain subjects of debate [1] . Although the permanent adhesive of the cyprid is the most poorly understood of the barnacle adhesives, it is also the system that resembles most closely the seemingly convergent adhesion mechanisms represented by the aforementioned groups of organisms. The presently accepted model for cyprid permanent adhesion, presented by Walker [16] , [17] , is that proteinaceous components of the adhesive are stored separately in the large (~120 μm longest length) kidney-shaped cement glands. Two cell types within the glands contain secretory granules with different morphologies (α and β granules) and differing compositions. Walker described that release, which we now know to be exocytosis, of the granules into a median collecting duct followed by mixing and expulsion of the adhesive under pressure: the material travelled down the antennules used for surface exploration, culminating in discharge through pores on adhesive disc of the 3rd antennular segment ( Fig. 1a,b ). The expressed adhesive then embedded the antennules and, depending on the surface, the two deposits of the adhesive (one from each antennule) often merged into one continuous plaque [18] ( Fig. 1c–e , Supplementary Movie 1 ). Having identified phenolic peptides and the enzyme polyphenoloxidase in the α-granules, Walker [16] surmised that separate adhesive components likely mix during release and cure via quinone tanning, forming a hard adhesive plaque. 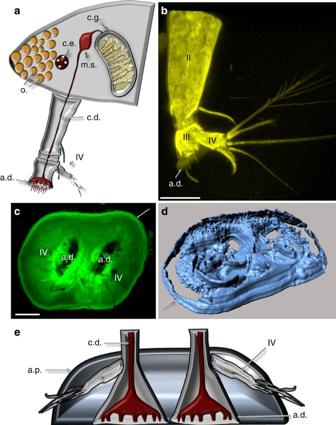Figure 1: Morphology of the cyprid adhesive apparatus and the expressed adhesive plaque. (a) A schematic of the anterior section of a barnacle cypris larva, with particular focus on the cementation apparatus: c.g., cement gland; m.s., muscular sac; c.d., cement duct; a.d., adhesive disc; o., oil bodies; c.e., compound eye; IV, fourth antennular segment, as per Walker17. (b) A confocal volume projection of a cyprid antennule labelled with a membrane dye showing the 2nd, 3rd and 4th segments of the antennule, the adhesive disc (a.d.) and setae of the 4th segment (IV). (c) Confocal micrograph of a cyprid adhesive plaque stained for proteins. Embedded within the plaque are the adhesive discs appearing as dark central regions and setae of the 4th segment. When viewed this way, the plaque appears to approximate the homogeneously proteinaceous, low-density structure originally described by Walker17, surrounded by a more protein-dense ‘skin’ (white arrow). (d) An isosurface rendering ofcshowing its 3D structure. (e) A sketch of the cyprid adhesive plaque as per Walker’s17description; adhesive plaque: a.p. Scale bars, ~20 μm (b–d). Figure 1: Morphology of the cyprid adhesive apparatus and the expressed adhesive plaque. ( a ) A schematic of the anterior section of a barnacle cypris larva, with particular focus on the cementation apparatus: c.g., cement gland; m.s., muscular sac; c.d., cement duct; a.d., adhesive disc; o., oil bodies; c.e., compound eye; IV, fourth antennular segment, as per Walker [17] . ( b ) A confocal volume projection of a cyprid antennule labelled with a membrane dye showing the 2nd, 3rd and 4th segments of the antennule, the adhesive disc (a.d.) and setae of the 4th segment (IV). ( c ) Confocal micrograph of a cyprid adhesive plaque stained for proteins. Embedded within the plaque are the adhesive discs appearing as dark central regions and setae of the 4th segment. When viewed this way, the plaque appears to approximate the homogeneously proteinaceous, low-density structure originally described by Walker [17] , surrounded by a more protein-dense ‘skin’ (white arrow). ( d ) An isosurface rendering of c showing its 3D structure. ( e ) A sketch of the cyprid adhesive plaque as per Walker’s [17] description; adhesive plaque: a.p. Scale bars, ~20 μm ( b – d ). Full size image The results of studies aiming to elucidate the nature of the permanent adhesive of cyprids have been ambiguous and often contradictory. Although Knight-Jones and Crisp [19] first presented evidence for quinone tanning, Hillman and Nace [20] obtained none. Hillman and Nace, on the other hand, presented the first evidence for a small quantity of lipid in the adhesive, an observation made by no other investigators. All early studies agreed that cyprid permanent adhesive is predominantly composed of protein, and this is consistent with what is known from studies of other marine bioadhesives. Walker’s original description of the adhesive plaque morphology [16] , based on transmission electron microscopy, noted three well-defined strata (layers 1, 2 and 3 from the outside in). With light microscopy, however, only two layers were visible—a low-density reticulum making up the majority of the plaque volume and a high-density external ‘skin’, both staining for protein [17] . Walker attributed the stratification in the original TEM micrographs to graded curing of the adhesive in the presence of an environmental catalyst; more recent observations using confocal laser-scanning microscopy (CLSM) have cast doubt upon that explanation, however [18] . Using CLSM, only two well-defined layers were visible: a central proteinaceous bulk and an external non-proteinaceous layer. Based upon these observations it is our view that the high-density external ‘skin’ observed by Walker under light microscopy was, indeed, the intermediate layer 2 in the original TEMs. We propose that layer 1 in Walker’s TEMs is the non-proteinaceous layer that was observed by Aldred et al . [18] This layer was probably removed during histological specimen processing in the early studies, which involved the use of ethanol, xylene, acetone and propylene oxide [16] , leaving only layer 2 as the outer skin. Based upon these recent insights and the apparent removal of layer 1 by organic solvents, we hypothesized that the true outer phase of the adhesive plaque is lipidaceous in nature. If so, this would constitute the first description of a lipid being used as a functional marine bioadhesive. To fully investigate this phase, the present study employs two-photon excited fluorescence microscopy (TPEFM), broadband coherent anti-Stokes Raman scattering (BCARS) microscopy, and CLSM, combined with a suite of fluorescent probes for lipids, lipopolysaccharides, proteins and phosphoproteins, to image cyprid adhesive plaques and excised cement glands. We further apply image analysis techniques, such as three-dimensional (3D) segmentation, polygonal mesh and isosurface generation to spatially delineate the two phases of the expressed adhesive. Here we show that the barnacle cyprid adhesive is a bi-phasic system; one phase composed of phosphoproteins and the other composed of lipids, and these phases are contained in two different granules within the cyprid cement glands. During adhesion the lipidaceous phase is released first into which the proteinaceous phase is secreted. We hypothesize that the outer lipidaceous phase creates a conducive environment for the curing and crosslinking of the proteins and protects the proteins from excessive hydration, spreading and bacterial degradation Two-photon microscopy of the cyprid adhesive plaques When adhesive plaques were stained for proteins, rendered images defined with great clarity, the high-density protein skin covering a low-density proteinaceous reticulum ( Fig. 1c,d , Supplementary Figs 1 and 2 and Supplementary Movie 1 ). High-magnification imaging of single embedded antennules, labelled specifically for primary amines, highlighted a void between the bulk protein core and bacterial growth on the true outer layer of the adhesive plaque, indicating a non-proteinaceous phase between the protein bulk and the ambient seawater ( Fig. 2a–f , Supplementary Movies 2 and 3 ). It is noteworthy that were it not for the visualization of bacterial growth on the true outer layer, this non-proteinaceous phase of the cyprid permanent adhesive would have been missed entirely. 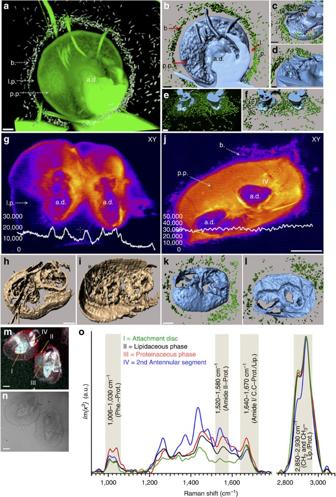Figure 2: Spatial arrangement of lipidaceous and proteinaceous components of the expressed adhesive. (a) CLSM volume projection of a single antennular adhesive plaque stained for proteins showing a clear void between the proteinaceous phase (green) and bacterial growth on the true outer phase of the adhesive plaque, which is not stained for proteins (b., bacteria; l.p., lipid phase; p.p., protein phase; a.d., adhesive disc). (b–d) Isosurface rendering ofaviewed from various angles. It is clear that proteinaceous phase (blue) and the bacterial growth (green) are separated by a material that does not stain for proteins. (e,f) Imaged during the adhesive secretion; the cyprid adhesive discs (blue) are embedded in a phase of the cyprid adhesive that did not stain for proteins but which accrued bacterial growth (green). (g) XY view from a TPEFM volume projection of the adhesive plaque embedding the paired antennules stained with lysochrome ORO. Relative fluorescence intensity units (RFU) plot (inset) shows lower intensity values when compared with the labelling of the proteinaceous phasej. (h,i) Isosurface renderings of the lipidaceous phase viewed from above (h) and beneath the plaque (i). The lipidaceous phase appears to entirely cover the bulk phase of the adhesive plaque, which is proteinaceous. (j) XY view from a TPEFM volume projection of an adhesive plaque stained for phosphoproteins shows that the bulk of cement plaque is phosphoproteinaceous and with much higher RFU as compared withg. (k,l) Isosurface renderings of phosphoprotein-stained plaque fromj, viewed from above (k) and beneath the plaque (l), shows that the bulk of the plaque is proteinaceous (blue) with bacterial growth (green) separated from the proteinaceous phase. (m–o) Pseudocoloured BCARS chemical image (m) with 500 nm lateral resolution taken at 30 ms per pixel acquisition times at 5 μm from coverslip surface. RGB image chemical contrast comes from total C-H stretch at 2,920 cm−1(red channel), the ratio of C-H to Amide III of 2,920:1,262 cm−1(green channel), and the ratio of C-H to nucleotide bases of 2,920:1,486 cm−1(blue channel). Bright-field image (n) from identical location as chemical image as well as spectra (o) obtained from individual pixels within BCARS chemical image to clarify distinct spectral differences between outer lipidaceous and inner regions of the adhesive plaque that are pointed to by arrows in chemical image. Scale bars (μm), 5 (a–c), ~2 (d), ~5 (e,f), ~20 (g,j), ~10 (h,i,k,l,) and 20 (m,n). Figure 2: Spatial arrangement of lipidaceous and proteinaceous components of the expressed adhesive. ( a ) CLSM volume projection of a single antennular adhesive plaque stained for proteins showing a clear void between the proteinaceous phase (green) and bacterial growth on the true outer phase of the adhesive plaque, which is not stained for proteins (b., bacteria; l.p., lipid phase; p.p., protein phase; a.d., adhesive disc). ( b – d ) Isosurface rendering of a viewed from various angles. It is clear that proteinaceous phase (blue) and the bacterial growth (green) are separated by a material that does not stain for proteins. ( e , f ) Imaged during the adhesive secretion; the cyprid adhesive discs (blue) are embedded in a phase of the cyprid adhesive that did not stain for proteins but which accrued bacterial growth (green). ( g ) XY view from a TPEFM volume projection of the adhesive plaque embedding the paired antennules stained with lysochrome ORO. Relative fluorescence intensity units (RFU) plot (inset) shows lower intensity values when compared with the labelling of the proteinaceous phase j . ( h , i ) Isosurface renderings of the lipidaceous phase viewed from above ( h ) and beneath the plaque ( i ). The lipidaceous phase appears to entirely cover the bulk phase of the adhesive plaque, which is proteinaceous. ( j ) XY view from a TPEFM volume projection of an adhesive plaque stained for phosphoproteins shows that the bulk of cement plaque is phosphoproteinaceous and with much higher RFU as compared with g . ( k , l ) Isosurface renderings of phosphoprotein-stained plaque from j , viewed from above ( k ) and beneath the plaque ( l ), shows that the bulk of the plaque is proteinaceous (blue) with bacterial growth (green) separated from the proteinaceous phase. ( m – o ) Pseudocoloured BCARS chemical image ( m ) with 500 nm lateral resolution taken at 30 ms per pixel acquisition times at 5 μm from coverslip surface. RGB image chemical contrast comes from total C-H stretch at 2,920 cm −1 (red channel), the ratio of C-H to Amide III of 2,920:1,262 cm −1 (green channel), and the ratio of C-H to nucleotide bases of 2,920:1,486 cm −1 (blue channel). Bright-field image ( n ) from identical location as chemical image as well as spectra ( o ) obtained from individual pixels within BCARS chemical image to clarify distinct spectral differences between outer lipidaceous and inner regions of the adhesive plaque that are pointed to by arrows in chemical image. Scale bars (μm), 5 ( a – c ), ~2 ( d ), ~5 ( e , f ), ~20 ( g , j ), ~10 ( h , i , k , l ,) and 20 ( m , n ). Full size image Figure 2e,f and Supplementary Movie 3 show only the outer phase of the plaque and the bacteria accumulated on it. Simultaneous labelling with various fluorescent probes specific to phosphoproteins and lipids indicated clearly the presence of a lipidaceous outer phase ( Fig. 2g–l , Supplementary Figs 3 and 4 and Supplementary Movies 4–7 ) and allowed detailed analysis of the respective phases of the adhesive plaque. The total volume of the lipid phase was considerably less than that of the protein phase, as evidenced by the difference in fluorescence intensities between lipid and protein-labelled adhesive plaques. The former formed only a thin outer layer around the proteinaceous core ( Fig. 2g–i ). BCARS imaging of the cyprid adhesive plaques Label-free BCARS chemical imaging of the adhesive plaques also showed a marked difference between spectra from these lipidaceous and inner proteinaceous phases. From the BCARS analysis, it was clear that one unique phase encircled the other from the interface through to the top of the plaque ( Fig. 2m–o and Supplementary Fig. 5 ). The thin outer layer possessed higher lipid content than other regions analysed, retaining a constantly higher ratio of CH 2 :CH 3 at the 2,875:2,930 cm −1 bands, but with a substantial decrease from the phenylalanine and amide I/II protein-specific vibrational modes at 1,006, 1,668 and 1,560 cm −1 , respectively [21] , [22] , [23] ( Fig. 2o ). The ratio between the CH 2 and protein-specific vibrational modes, or lipid:protein ratio, is indicative of local concentrations of the two species in biological systems [24] , [25] . The thin layer surrounding the bulk material was, therefore, unambiguously lipid-containing. In contrast, the central bulk of the adhesive contained a much higher concentration of protein-specific chemical moieties than that of even the surrounding tissue (for example, antennules and adhesive disc) of the cyprid. Functional imaging of the cyprid cement glands The presence of a functional lipid component in the adhesive necessitated a re-examination of the adhesive storage apparatus, that is, the cyprid cement glands and the contents of their two cell types. Previous histological investigations failed to detect a significant lipid component in either the α- or β-granules owing, perhaps, to the use of harsh organic solvents in traditional histological preparations. In fact, a 2006 study [26] questioned the existence of a second granule type. Not only is this assertion shown here to be unfounded but the images of toluidine blue-stained sections in the 2006 paper are themselves indicative of two granule types, one of which appeared to be lipid (cyan in colour). In the present study, under physiological conditions and without the use of harsh organic solvents, we present conclusive evidence of two granule types, stored separately in large columnar cells within the cement glands ( Fig. 3a and Supplementary Fig. 2d ). Our observations, however, depart somewhat from those of Walker [16] in relation to the biochemistry of the adhesive constituents and the arrangement of the cell types. Whereas α-granules stained positively for protein, as described previously, and constitute the bulk of the cement gland volume ( Fig. 3c,g,h , Supplementary Fig. 6 , Supplementary Movie 8 ), β-granules contain negligible protein and stained positively for lipids ( Fig. 3b,d–f , Supplementary Fig. 7 and Supplementary Movie 9 ). We have also shown that the α-granules are primarily composed of phosphoproteins. Walker’s arrangement of β-granule-containing cells at the dorsal and ventral extremes of the gland seems to be another artefact of physical sectioning of specimens. Instead, we observed cells containing β-granules along the entire length of the gland, but confined to the lower half closest to the median collecting duct ( Fig. 3e , Supplementary Fig. 7 and Supplementary Movie 9 ). Although cement gland cells contain only one granule type, of either proteinaceous or lipidaceous composition, the proximity of the β-granules to the median collecting duct would support their being exocytosed first, followed by the α-granules. This hypothesis was also supported by the fact that during initial stages of adhesive release, the released adhesive did not fluoresce when labelled with protein-specific stains, while it showed strong fluorescence when labelled with lipid-specific stains, implying a sequential release of adhesive components from the cement glands where the lipid phase is released first. The natural process of exocytosis has never been observed in cyprids, although artificial stimulation using catecholamines has been achieved [9] , [27] ( Supplementary Movie 10 ). 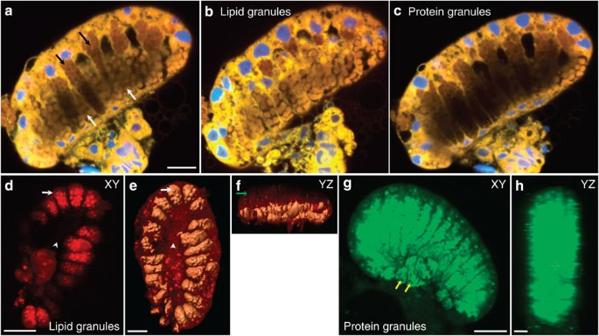Figure 3: Spatial arrangement of lipidaceous and proteinaceous adhesive granules within the cyprid cement gland. Using a combination of lipid-specific (FM 1-43 FX) and protein-specific (fluoresceinamine) dyes we confirm: (a) the presence of two granule types within separate columnar cells of the cement gland; lipidaceous granules (white arrows) and proteinaceous granules (black arrows) in this confocal micrograph. Cell nuclei are blue. (b) Lipidaceous granule-containing cells are present along the entire length of the gland and are not restricted to the dorso-ventral extremes, with their contents concentrated closest to the median cement-collecting duct. (c) Proteinaceous granule-containing cells are also distributed throughout the length of the gland. Lipidaceous granules appear to be larger than the proteinaceous granules and are packed more loosely. (d) TPEFM volume projection of cement gland stained with Nile-Red, showing that the lipidaceous granules (white arrow) in the lipid granule-containing cells are present only in the lower ventral half of the gland, closest to the median cement-collecting duct (arrow head). (e) Isosurface rendered view of the lipidaceous granule-containing cells superimposed onto the volume projection of the gland. (f) YZ orthogonal view of the Nile-Red-labelled cement gland. Since Nile-Red does not label the proteinaceous granules, the bulk of the cement gland appears empty (green arrow). (g) TPEFM volume projection of a cement gland stained specifically for phosphoproteins showing that proteinaceous granules constitute the bulk of the gland; also seen in YZ orthogonal view inh. Lipidaceous granules present around the collecting duct are not labelled by the phosphoprotein stain and appear as vacuoles (yellow arrow). Also seeSupplementary Figs 6 and 7. Scale bars (μm), ~20 (a–c,d,e), ~30 μm (g,h). Figure 3: Spatial arrangement of lipidaceous and proteinaceous adhesive granules within the cyprid cement gland. Using a combination of lipid-specific (FM 1-43 FX) and protein-specific (fluoresceinamine) dyes we confirm: ( a ) the presence of two granule types within separate columnar cells of the cement gland; lipidaceous granules (white arrows) and proteinaceous granules (black arrows) in this confocal micrograph. Cell nuclei are blue. ( b ) Lipidaceous granule-containing cells are present along the entire length of the gland and are not restricted to the dorso-ventral extremes, with their contents concentrated closest to the median cement-collecting duct. ( c ) Proteinaceous granule-containing cells are also distributed throughout the length of the gland. Lipidaceous granules appear to be larger than the proteinaceous granules and are packed more loosely. ( d ) TPEFM volume projection of cement gland stained with Nile-Red, showing that the lipidaceous granules (white arrow) in the lipid granule-containing cells are present only in the lower ventral half of the gland, closest to the median cement-collecting duct (arrow head). ( e ) Isosurface rendered view of the lipidaceous granule-containing cells superimposed onto the volume projection of the gland. ( f ) YZ orthogonal view of the Nile-Red-labelled cement gland. Since Nile-Red does not label the proteinaceous granules, the bulk of the cement gland appears empty (green arrow). ( g ) TPEFM volume projection of a cement gland stained specifically for phosphoproteins showing that proteinaceous granules constitute the bulk of the gland; also seen in YZ orthogonal view in h . Lipidaceous granules present around the collecting duct are not labelled by the phosphoprotein stain and appear as vacuoles (yellow arrow). Also see Supplementary Figs 6 and 7 . Scale bars (μm), ~20 ( a – c , d , e ), ~30 μm ( g , h ). Full size image Based upon our observations, we propose a novel mechanism for the permanent adhesion of the barnacle cypris larva in which a lipidaceous primer, stored in the β-granules, is released first. We hypothesize that this material displaces water from the interface creating an environment conducive to the curing of a subsequent proteinaceous component, released by the α-granules ( Fig. 4a,b ). This environment would not be anhydrous per se , and need not be, since hydrated coacervate-like bioadhesives are perfectly adapted for adhesion to hydrated interfaces [14] . Rather, we suggest that excessive and uncontrolled dissolution of the adhesive is prevented by a pre-existing outer layer of lipid. The solvation shell created by the long, non-polar, hydrocarbon chains in the lipids will reduce the entropy of the plaque at the lipid–water interface, excluding water and preventing excessive hydration of the protein phase. It was also shown previously [18] that this outer phase exerts a controlling effect on the spreading of the inner phase, depending on the chemical nature of the substratum, and may therefore be fundamental to the regulation of adhesive spreading. 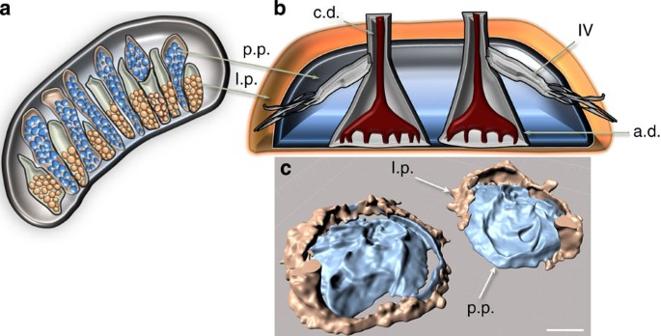Figure 4: A new model for the permanent adhesion of barnacle cyprids. (a) A schematic of the sagittal section of the cement gland. A lipidaceous precursor material (l.p.) is released from the lipid granule-containing cells (orange) closest to the cement collecting duct. Subsequently, the contents of the protein granule-containing cells (blue) are released into the lipidaceous phase, already delivered to the surface. (b) A lipidaceous phase (orange) that surrounds the proteinaceous core (blue) of the adhesive plaque is the result, and is even present at the adhesive interface. (c) TPEFM isosurface rendered volume projection showing two individual cyprid cement plaques, each embedding a single antennule, labelled for proteins (blue) and lipids (brown). l.p., lipidaceous phase; p.p., proteinaceous phase. Schematics not drawn to scale. Scale bars, ~20 μm (c). Figure 4: A new model for the permanent adhesion of barnacle cyprids. ( a ) A schematic of the sagittal section of the cement gland. A lipidaceous precursor material (l.p.) is released from the lipid granule-containing cells (orange) closest to the cement collecting duct. Subsequently, the contents of the protein granule-containing cells (blue) are released into the lipidaceous phase, already delivered to the surface. ( b ) A lipidaceous phase (orange) that surrounds the proteinaceous core (blue) of the adhesive plaque is the result, and is even present at the adhesive interface. ( c ) TPEFM isosurface rendered volume projection showing two individual cyprid cement plaques, each embedding a single antennule, labelled for proteins (blue) and lipids (brown). l.p., lipidaceous phase; p.p., proteinaceous phase. Schematics not drawn to scale. Scale bars, ~20 μm ( c ). Full size image Our evidence suggests that the lipid phase is released first, followed by the proteinaceous second phase. While it is conceivable that the two components could be released in a gradient, beginning with a high concentration of the lipidaceous phase and ending with the proteinaceous phase, the clear demarcation between phases observed by Aldred et al. [18] suggests that this is unlikely. Established theory, based upon the observations of Walley [28] , presents an alternative and seemingly inaccurate hypothesis whereby adhesive components are mixed, post-exocytosis, in a muscular sack ( Fig. 1a ) before release to the surface. Walley originally proposed this only as a hypothesis based upon the available evidence but the process was never observed in vivo . Mixing of the components, followed by release and subsequent phase-separation ex vivo is precluded by our observations early in the process of cement release, where only lipid was evident on the surface. As the proteinaceous bulk of the adhesive is released into the lipidaceous phase, the former becomes concentrated at the interface between the two materials, resulting in a protein-dense interphase region. From our observations it is also apparent that, being rich in proteins, the proteinaceous phase would serve as a nutrient source for benthic bacteria and that the lipid phase may have a protective role, reducing bacterial biodegradation as the proteins cross link and cure. The result is a solid proteinaceous core that embeds the antennules and maintains the cohesive structure of the plaque ( Fig. 4c ). This phase is surrounded and possibly even adhered to the surface by the lipid-based primer. Lipid was often observed as faint fluorescence between the adhesive plaque and the surface ( Fig. 4b ), but with a signal insufficient to allow isosurface rendering. Although lipid is the major component of the putative primer, the true composition of the material is likely lipoprotein and/or lipopolysaccharide ( Supplementary Fig. 7i,j ). As the outer phase is sufficiently robust to survive days to weeks in the marine environment, we do not exclude a degree of crosslinking of functional groups, nor do we discount the possibility of any proteins in the external phase serving in the initiation and maintenance of adhesion to surfaces. AFM was used to demonstrate both hardening of the outer phase over the course of an hour or so post-secretion [29] and the time-limited susceptibility of the adhesive plaque to attack by protease enzymes [30] . The vanishingly small quantity of adhesive available for collection per cyprid, and even smaller amounts of the individual phases, severely limit the use of conventional analytical techniques to elucidate the nature of cyprid adhesive. Surprisingly, while describing larval cement in another genus of barnacles, Darwin [11] noted that ‘...the cement, or part at least, comes out of the ultimate segment of the antennae, in the shape of one tube, within another tube of considerable diameter and length’, and it is our understanding that this refers to the ‘fried egg’-like appearance of the adhesive plaque in low magnification microscopy. This optical effect may now be assigned to the presence of two concentrically arranged components of differing composition. Whether or not this type of bi-phasic mechanism is more widespread in marine bioadhesives is unclear, as the role of lipids in adhesion has rarely been investigated. ATR-FTIR peaks corresponding to lipid esters were observed at the adhesive interface of mussel byssal threads [31] , but little relevant information is available in the literature regarding putative lipid fractions of adhesive secretions from other organisms. Having previously received scant attention in the literature, it is our view that lipids, lipoproteins and/or lipopolysaccharides could play an important functional role in the adhesive systems of other marine organisms too. Their role is well-established in the tarsal adhesive secretions of terrestrial arthropods [32] , [33] , for example. Importantly, if we accept Darwin’s and, later, Walker’s hypotheses that the cyprid cement glands ultimately constitute the adult cement apparatus in barnacles (recently supported by ref. 34 ), these observations will also have important repercussions for our understanding of adult barnacle adhesion and practical applications thereof. Cyprid culture Barnacle larval culture was carried out at Duke University Marine Laboratory in Beaufort, North Carolina, USA. Balanus amphitrite Darwin (1,854) (= Amphibalanus amphitrite ) nauplii (planktonic feeding stage) were obtained from field-collected adults and were incubated for 4 days at 27–28 °C. Larvae were raised on a diet of excess Skeletonema cosatum . Following 4 days of incubation, cyprids (settlement-stage larvae) were separated from the culture through a series of fine mesh filters and were isolated, cleaned and then shipped to Clemson University via overnight carrier at 6–8 °C. Larvae were maintained at 6–8 °C until use in experiments [18] , [35] . Sample preparation for staining cyprid cement plaques Cyprids maintained at 6–8 °C were acclimated to room temperature (RT). Cyprids were then deposited on #1.5 borosilicate coverglass (Thermo-Fisher) in a 1-ml drop of artificial seawater (ASW) (33‰) and allowed to settle at 23 °C in a humidified incubator for 6–8 h (ref. 18 ). Permanently attached cyprids that had not metamorphosed into juvenile barnacles were subjected to the various staining procedures described below. Cyprid cement gland dissection Cyprid cement glands were dissected as described previously [35] , [36] . Briefly, the dissections were carried out on #1.5 borosilicate coverglass (Thermo-Fisher) with the aid of a Nikon SMZ 800 stereo-microscope. Cyprids were relaxed by adding a 7.5% (w:v) MgCl 2 drop-wise to Petri dishes containing cyprids in ASW. Once the cyprids were relaxed, the adductor muscle at the junction of the bivalve carapace was severed using acid-etched tungsten micro-needles (Fine Science Tools Inc., No. 10130-10, Foster City, CA, USA). Cement glands were then dissected out, separated and cleaned from associated tissue debris, brain, eyes and antennules. The cement glands were also subjected to staining procedures. Nile Red staining for lipids Nile Red is a lipophilic stain that exhibits environment-sensitive fluorescence [37] . It is not fluorescent in aqueous media but is intensely fluorescent in lipid-rich environments [38] . A 1 mM stock solution of Nile Red (Sigma-Aldrich cat no. N-3013) was prepared in DMSO. From the stock, a working solution at 800 nM was prepared by dilution in phosphate-buffered saline (PBS). Cement glands and/or plaques on coverglass were placed in Petri dishes containing 4% formaldehyde solution freshly prepared from paraformaldehyde in PBS and allowed to fix for 30 min at RT. Samples were then washed twice with PBS for 5 min each on an orbital shaker to remove the fixative. Glands and plaques on coverglass were immersed in Nile Red staining solution for 15 min at RT, followed by two washes for 5 min each with PBS on the orbital shaker to remove excess dye. A second #1.5 coverglass was placed gently on top of the coverglass containing specimen and a drop of PBS. The two coverslips were slightly separated and temporarily sealed using silicone grease (General Electric). Two-photon excitation and emission wavelengths: ex755 nm, band-pass emission filter at 535/50 nm. Oil-Red-O staining for lipids For Oil-Red-O staning [39] , [40] , cement glands or plaques on coverglass were fixed with formaldehyde as described above and immersed in Oil-Red-O (ORO; Sigma-Aldrich cat no. O0625) staining solution for 20 min, followed by washing twice with PBS for 5 min each on an orbital shaker. ORO staining solution (100 ml) was prepared by adding 40 ml of dH 2 0 to 60 ml of 12 mM solution of ORO in 100% isopropanol. The ORO-staining solution was allowed to stabilize at RT for 20 min and then filtered through a 0.2-μm filter (Nalgene). Coverglass were prepared for imaging as described above. Two-photon excitation and emission wavelengths: ex755 nm, band-pass emission filter at 535/50 nm. Staining for lipopolysaccharides Glands and/or adhesive plaques were subjected to lipopolysaccharide staining using Pro-Q Emerald stain (cat no. P20495, Life Technologies, Carlsbad, USA) [41] . Although the Pro-Q Emerald manufacturer’s protocol is designed for staining polyacrylamide gels, it was modified in this case to stain glands and adhesive plaques. Briefly, formaldehyde-fixed and PBS-washed glands and/or plaques were treated with the carbohydrate-oxidizing solution (3% acetic acid and periodic acid solution, provided with the kit) for 15 min, washed twice with PBS for 5 min each on an orbital shaker and then incubated with the Pro-Q Emerald staining solution for 30 min. This was followed by two PBS washes for 5 min each on an orbital shaker. Coverglass were prepared for imaging as described above. Two-photon excitation and emission wavelengths: ex800 nm, band-pass emission filter at 535/50 nm. Differential staining with lipid and protein dyes Cement glands and/or adhesive plaques on coverglass were stained with a solution of the lipid membrane dye FM 1-43 FX (Life Technologies) prepared in DMSO in ASW at a final concentration of 5 mM for 10 min. Specimens were then washed twice with ASW for 5 min each on an orbital shaker and fixed with freshly prepared PBS buffered 4% formaldehyde for 30 min. Fixed specimens were washed with PBS twice for 5 min each on an orbital shaker and then incubated with a 1.4 mM solution of fluoresceinamine in PBS for 30 min. Fluoresceinamine binds to primary amines in proteins [18] . Specimens were washed twice with PBS and coverglass prepared for imaging as described above. Phosphoprotein staining Although the manufacturer’s protocol for Pro-Q Diamond phosphoprotein stain (cat no. MPP33300, Life Technologies) [42] is optimized for staining SDS-polyacrylamide gels, it was modified to stain cement glands and adhesive plaques. Briefly, cement glands and adhesive plaques were fixed with formaldehyde, as described previously. PBS-washed specimens were incubated with the Pro-Q Diamond staining solution for 60 min at RT while gently shaking on an orbital shaker. Following staining, the specimens were washed with PBS three times for 10 min each while on the orbital shaker. Coverglass were prepared for imaging as described above. Two-photon excitation and emission wavelengths: ex800 nm, band-pass emission filter at 610/75 nm. Coomassie blue staining of adhesive plaques Formaldehyde-fixed and PBS-washed plaques were stained with 0.01% Coomassie Brilliant Blue R-250 (Sigma) in 50% methanol and 10% acetic acid for 1 h at RT. Following staining, plaques were de-stained with 40% methanol and 7% acetic acid for 10 min on an orbital shaker followed by a gentle rinse with PBS and 10 min PBS wash on an orbital shaker. Two-photon excitation and emission wavelengths: ex700 nm, band-pass emission filter at 535/50 nm. Noradrenaline-induced exocytosis of cement granules Cyprid cement glands were dissected on coverglass as described above. The coverglass were then placed on the microscope stage and a 20 μM solution of noradrenaline, prepared in 0.2 μm filtered ASW, was added drop-wise to immerse the glands. An image series was recorded at multiple time points in differential interference contrast mode. Before carrying out any of the staining methods described above, unstained specimens (adhesive plaques and cement glands) were checked for auto-fluorescence at excitation and emission wavelengths used in the experiments using both single-photon CLSM and two-photon exited fluorescence microscopy. Control samples, which were carried through the staining procedures, but without the addition of stains, were also imaged to check for non-specific fluorescence and auto-fluorescence. Neither the unstained nor the control samples exhibited auto-fluorescence in the emission wavelengths used for the assays. Single-photon CLSM CLSM on cement glands and/or plaques was performed as described previously [35] , [43] . Briefly, specimens were imaged on a Nikon Eclipse TiE inverted microscope (Nikon, Melville, NY, USA), equipped with a C1Si spectral confocal scan head, following laser lines, 405, 457, 476, 488, 514, 561, 638 nm and appropriate band-pass filter sets for the excitation and emission wavelengths of fluorophores used. Imaging was carried out using Nikon CFI Plan Fluor × 20, 0.45 numerical aperture (NA) and Nikon CFI Plan Apo × 60, 1.2 NA objectives. The microscope was also equipped with a CoolSnap-HQ2 monochrome CCD camera (Photometrics, USA) and a Lambda 10-3 Motorized filter wheel (Sutter Instruments, Novato, California, USA) [44] . Multi-channel time lapse of noradrenaline-induced cement gland exocytosis was imaged by setting up a ‘time lapse’ routine in Nikon NIS Elements software controlling the microscope that acquired images automatically over a defined period of time. Two-photon excited fluorescence microscopy TPEFM was performed by coupling a mode locked beam of a Ti:Saphire oscillator at 140 fs pulses at 80 MHz repetition rate (Chameleon Ultra-II, Coherent, Santa Clara, CA, USA) to a Movable Objective Microscope (Sutter Instruments, Novato, CA, USA) [45] , [46] . The laser intensity delivered to the microscope was controlled using a pockel cell, model 302RM driver and a model 350-80-LA-02 EO modulator (Conoptics, Danbury, CT, USA). The laser beam was raster-scanned in the microscope via a pair of galvanometric scanners (Cambridge Technologies, MA, USA) and projected onto a back aperture of a Nikon CFI Apo LWD × 25, 1.1 NA water immersion objective through a scan and tube lens. The four-channel non de-scanned detector set-up consisted of four GaAsP photomultiplier tubes H7422P40-MOD (Hamamatsu, Middlesex, NJ, USA) with appropriate band pass filters for excitation and emission wavelengths of the fluorophores used in the experiments. The microscope’s X,Y,Z movements, laser intensity modulation by the pockel cell and data acquisition were carried out using MScan software (Sutter Instruments). BCARS microscopy Coherent anti-Stokes Raman scattering [47] is used as an analytical tool and an imaging contrast mechanism in the realms of materials and biological sciences [47] , [48] , [49] , [50] . BCARS contributes to the suite of traditional CARS capabilities by providing improved chemical selectivity and sensitivity over a 3,000 cm −1 spectral range. The ability of BCARS to chemically image complex samples for obtaining a broad spectral signal at very short image acquisition times (<30 ms per pixel of blue-shifted light) and at high spatial resolution (<1 μm 3 per spectral voxel) arises entirely from CARS being a nonlinear, third-order optical process where, ω anti-Stokes = ω Probe + ω Pump − ω Stokes (refs 51 , 52 , 53 , 54 ). As a result, BCARS has the ability to non-invasively measure localized Raman signals at high speeds without auto-fluorescence of biological samples and in 3D sample space free of any sample preparation and labelling. The coherent Raman (BCARS) microscope is detailed in the schematic diagram in Supplementary Fig. 8 . In detail, the output (70-fs pulses centred at 830 nm and a 80 MHz repetition rate) from a single Ti:Sapphire oscillator (MaiTai-DeepSee, Spectra Physics, Santa Clara, CA, USA) was split into two separate beams: one for the pump/probe transitions and other for the Stokes transitions. The bandwidth of one beam for the pump and Stokes transitions (narrowband pulse) was reduced by adjusting the slit width in a 4- f dispersionless filter to 8 cm −1 at full-width half-maximum, with the centre wavelength at 830 nm. The other beam was sent through a photonic crystal fiber (Crystal Fiber- Femtowhite 800, NKT Photonics, Morgnaville, NJ, USA) for supercontinuum generation to produce a spectrally broad (850–1,200 nm) pulse and then collimated using a parabolic mirror. The two beams were then collinearly combined before entering into the side port of an inverted microscope (Olympus IX71, Olympus, Allentown, PA, USA). The beam was focused onto the sample using a × 40, 0.95 NA objective lens (Olympus) for a lateral resolution spot size of ~0.5 μm. The average power at the focal point of the beam was ~14 mW. The scattered light was collected by a × 60, 0.8 NA objective lens (Olympus) and then passed through an 830 nm notch filter and an 810 nm short-pass filter to remove the excitation light. After filtering, the blue-shifted BCARS signal was introduced into a spectrograph (SP-2300, Acton with 600 lines/mm grating) and measured with a charged-coupled device (CCD, DU920-BR-DD, Andor, South Windsor, CT, USA). The exposure time on the CCD was 30 ms per sample spatial location over a spectral region of 800–3,400 cm −1 across 1,024 pixels of the CCD chip. Images were produced by scanning the sample laterally and axially in 0.5 μm increments. Image acquisition and initial analysis were performed using a custom-developed LabView (LabView 2011, National Instruments, Austin, TX, USA) programme. BCARS spectral data processing included cosmic ray spike removal, spectral phase retrieval using the time-domain Kramers–Kronig approach to extract the resonant Raman signal, and baseline detrending using a cubic-spline algorithm [55] , [56] . Data analysis and visualization for CLSM and TPEFM Optical Z-sections (Z-series) collected using TPEFM were first converted to multipage TIFF (tagged image file format) files using Mview image analysis programme (Sutter Instruments). Multi-page TIFFs were then converted to Image Cytometry Standard file formats (.ics) using NIS Elements (Nikon). Image files in .ics formats from CLSM and TPEFM were analysed using NIS Elements and Imaris (Bitplane, Zurich, Switzerland) data analysis and visualization software. Two-dimensional images were exported and saved in TIFF format and assembled into a figure panel using PowerPoint (Microsoft). 3D volume renderings created in NIS Elements and Imaris were exported as .AVI files for Supplementary Movies . 3D polygonal mesh surface renderings were created from the confocal and two-photon data sets using Imaris. Briefly, Imaris allows segmentation of the data sets and use of algorithms, like Marching Cubes, to extract a polygonal mesh of an isosurface from voxels of the 3D data set. Adobe Photoshop CS5 was only used for creating Supplementary Fig. 2 . For that figure, images were inverted using the ‘invert’ function in Photoshop and grayscale gradient mapping was assigned to the images using the ‘gradient map’ function. Brightness, contrast and gamma were then adjusted for the images and the figure panel was assembled using Microsoft PowerPoint. Certain equipment, instruments or materials are identified in this paper in order to adequately specify the experimental details. Such identification does not imply recommendation by the National Institute of Standards and Technology (NIST) nor does it imply the materials are necessarily the best available for the purpose. How to cite this article: Gohad, N. V. et al. Synergistic roles for lipids and proteins in the permanent adhesive of barnacle larvae. Nat. Commun. 5:4414 doi: 10.1038/ncomms5414 (2014).